Towards evidence-based response criteria for cancer immunotherapy 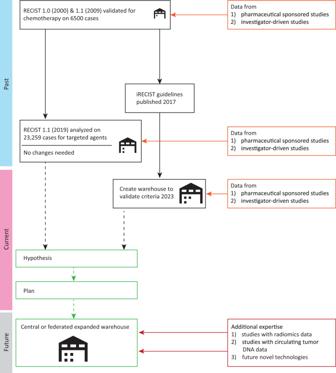Fig. 1: Evolution of RECIST. This figure shows the activities regarding the development of RECIST in the past (in blue), currently (in pink) and to be expected in the future (in gray). The increasing size of the warehouse represents the increasing number of data in the warehouse. RECIST has become the widely adopted standard criteria used in early clinical trials of novel agents for solid tumors to determine the response-based endpoints, response rate, duration of response, and progression-free survival. Its validity has been confirmed for cytotoxic chemotherapy and for targeted therapy using shared data on patients enrolled in both academic and industry-sponsored clinical trials. Proposed criteria, iRECIST, have been incorporated as an exploratory endpoint into many clinical trials of immunotherapeutic agents in order to capture unusual patterns of response that can occur with these agents. Validation of iRECIST will require sharing clinical trial data from patients receiving immunotherapy agents. These analyses will look at the data in aggregate, without regard to the specific agent used, and will not compare agents. The analyses will be performed simply to confirm the usefulness of iRECIST as a surrogate endpoint in trials of immunotherapy agents and to see if iRECIST adds more than standard RECIST criteria in this situation. If so, then iRECIST could be adopted as the standard response assessment for immunotherapeutic agents. It can be envisioned that novel imaging and imaging analyses, as well as circulating tumor DNA approaches for response criteria, might be developed and included in the future.